Momentum-dependent multiple gaps in magnesium diboride probed by electron tunnelling spectroscopy The energy gap is the most fundamental property of a superconductor. MgB 2 , a superconductor discovered in 2001, exhibits two different superconducting gaps caused by the different electron–phonon interactions in two weakly interacting bands. Theoretical calculations predict that the gap values should also vary across the Fermi surface sheets of MgB 2 . However, until now, no such variation has been observed. It has been suggested that two gap values were sufficient to describe real MgB 2 samples. Here we present an electron tunnelling spectroscopy study on MgB 2 /native oxide/Pb tunnel junctions that clearly shows a distribution of gap values, confirming the importance of the anisotropic electron–phonon interaction. The gap values, and their spreads found from the tunnel junction measurements, provide valuable experimental tests for various theoretical approaches to the multi-band superconductivity in MgB 2 . There has been a surge of interest in multi-band superconductivity owing to its existence in MgB 2 (refs 1 , 2 , 3 , 4 ), iron-based superconductors [5] , and other superconducting materials [6] , [7] , [8] . The crystal structure of MgB 2 is formed by layers of honeycombed boron atoms intercalated with magnesium atoms located above the centre of the boron hexagons. The boron s , p x , and p y orbitals form quasi-two-dimensional σ bands, which couple strongly to the in-plane boron E 2 g phonon mode and results in the formation of superconducting σ gaps of about 7 meV. The boron p z orbit forms the three-dimensional π bands that have a much weaker coupling to the E 2 g mode, leading to π gaps of about 2 meV. There is a finite coupling between the π and σ bands, and both gaps vanish at a common T c . Besides the two widely observed gaps [9] , [10] , [11] , [12] , first-principles calculations taking into account the fully anisotropic electron–phonon interaction predict that there should also be an intraband anisotropy within the σ and π gaps [1] , [2] . In an earlier work Choi et al . solved the Eliashberg equation in the clean limit, using an anisotropic electron–phonon interaction λ( k , k ′), and found an energy gap Δ( k ) that spreads between 1.2 and 3.7 meV for the π bands and from 6.4 to 7.2 meV for the σ bands [1] , [13] . Later, direct first-principles calculations by Floris et al ., using superconducting density functional theory without any semi-phenomenological parameters for the Coulomb repulsion, confirmed the existence of the anisotropy [2] . However, experimental evidence for a distribution of gap values, beyond just two values, has been lacking. Mazin et al . have suggested that the gap distribution cannot be resolved owing to the effects of intraband scattering [14] . Electron tunnelling spectroscopy probes the quasiparticle density of states (DOS) in a superconductor, and thus provides the most direct measurement of the superconducting energy gap [15] . Previously, we have reported MgB 2 /native oxide/Pb tunnel junctions with bottom electrode being c -axis-oriented MgB 2 film grown by hybrid physical–chemical vapour deposition (HPCVD) on (0001) single crystal 6H-SiC substrate [16] . The predominant structure in the tunnelling spectra of these junctions is from the π gap as the σ carriers are mostly confined to the a – b planes. When the a – b planes of the bottom MgB 2 electrode are exposed for electron tunnelling, such as in MgB 2 films on MgO (211) substrate, where the c axis is tilted by 19.5° away from the film normal [17] , contributions from the σ gap can also be observed. These tunnel junctions enable us to study both the π and σ gaps of MgB 2 . In this study, we performed electron tunnelling spectroscopy measurements using MgB 2 /native oxide/Pb tunnel junctions made from HPCVD-grown MgB 2 films on MgO (211), SiC (0001), and c -axis-8°-tilted SiC substrates. The observed conductance peaks due to the σ and π gaps show fine structure, from which we derived the distribution of gap values within the two gaps. Most likely, the cleanliness of the MgB 2 electrode and the high-quality MgB 2 /oxide interface made the observation possible, because increased scattering in the MgB 2 electrode and a high junction resistance were found to smear out the fine structure. The experimentally obtained gap distribution is in agreement with the first-principles calculations. 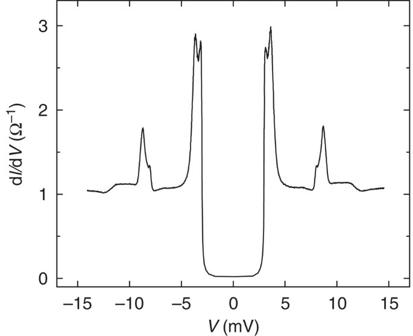Figure 1: Tunnelling spectrum of a MgB2/native oxide/Pb junction at 1.8 K. Both the π-gap feature and the σ-gap feature show subtle peak structure. Tunnelling spectra The tunnelling conductance d I /d V versus voltage V for a MgB 2 /native oxide/Pb junction on MgO (211) at T =1.8 K is shown in Figure 1 . Two sets of conductance peaks are seen in the spectrum. The peaks around±3.5 mV correspond to ±(Δ π +Δ Pb ), and the peaks around±8.5 mV to±(Δ σ +Δ Pb ), where Δ π , Δ σ , and Δ Pb denote the superconducting gaps in the MgB 2 π band, MgB 2 σ band, and Pb, respectively. The spectrum can be fitted to the standard tunnelling equation, assuming that the total normalized DOS N (ɛ) is a linear combination of the contributions from the π and σ bands ( N π and N σ , respectively), that is, The coefficient r represents the contribution of the π band to the DOS, which is 89% for this junction [17] . It can be seen that both the π and σ peaks are not simple, smooth ones, but exhibit fine structure. Figure 1: Tunnelling spectrum of a MgB 2 /native oxide/Pb junction at 1.8 K. Both the π-gap feature and the σ-gap feature show subtle peak structure. Full size image Subtle gap features are not caused by Pb To rule out the contribution of the Pb energy gap to the fine structure, we made Pb/PbO/Pb junctions with Pb films grown under the same conditions as the MgB 2 /native oxide/Pb junctions. 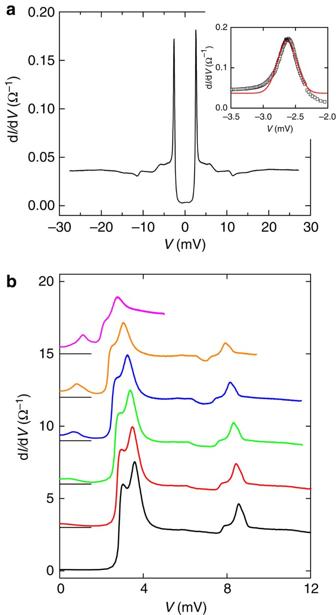Figure 2: The subtle gap peak structure is not caused by Pb. (a) Tunnelling spectrum of a Pb/PbO/Pb junction atT=4.2 K. (inset) The single peak at about −2.6 mV corresponds to twice the average superconducting gap of Pb. The experimental data (squares) are fit by a Gaussian function (line). (b) The tunnelling spectra of a MgB2/native oxide/Pb junction atT=4.2, 5.0, 5.5, 6.0, 6.5 and 7.0 K (curves from bottom to top). The curves are shifted vertically for clarity with horizontal bars indicating zero conductance. A typical tunnelling spectrum is shown in Figure 2a . The sharp peaks at V =±2.62 mV correspond to the double gap. The Gaussian fit in the inset to Figure 2a shows only one single peak with full-width-at-half-maximum (FWHM) around 0.29 mV, indicating an average energy gap of about 1.31±0.01 meV at 4.2 K. This also suggests that the resolution of our tunnelling measurement at 4.2 K is better than 0.29 mV. Figure 2b shows the tunnelling spectra of another MgB 2 /native oxide/Pb junction on MgO (211) at temperatures in the range of 4.2 to 7.0 K, over which the gap of Pb changes substantially. Although the conductance peaks shift to lower voltages when the temperature increases, owing to the temperature dependence of the Pb gap, the basic fine structure does not change. Thus the fine structure can be definitively attributed to MgB 2 , as the MgB 2 gaps are insensitive to temperature in this range ( T < T c /2). Figure 2: The subtle gap peak structure is not caused by Pb. ( a ) Tunnelling spectrum of a Pb/PbO/Pb junction at T =4.2 K. (inset) The single peak at about −2.6 mV corresponds to twice the average superconducting gap of Pb. The experimental data (squares) are fit by a Gaussian function (line). ( b ) The tunnelling spectra of a MgB 2 /native oxide/Pb junction at T =4.2, 5.0, 5.5, 6.0, 6.5 and 7.0 K (curves from bottom to top). The curves are shifted vertically for clarity with horizontal bars indicating zero conductance. Full size image Deconvolution of tunnelling spectra Because the normalized quasiparticle DOS of Pb is given by the BCS expression where Δ Pb is 1.35 meV at 1.8 K, we can derive the DOS of MgB 2 by deconvoluting the tunnelling I – V curve using an approach first used by Blamire [18] . We do not consider the phonon structure of Pb at around 7 meV and 11 meV caused by the strong electron–phonon couplings [19] , because their effects are negligible compared with the contributions owing to the energy gaps. The tunnelling current of a MgB 2 /native oxide/Pb junction can be expressed as where N MgB2 is the MgB 2 DOS, e is the electron charge, and f is the Fermi distribution function [15] . At low temperatures, the region Δ m / e < u < V –Δ Pb / e dominates the integration (greater than 99% for V >2.8 mV at T =1.8 K), where Δ m ~1.3 meV is the smallest gap value for MgB 2 . The points of the MgB 2 DOS are sequentially obtained from the tunnelling spectrum shown in Figure 1 by discretizing the integrations over successively larger ranges [18] . 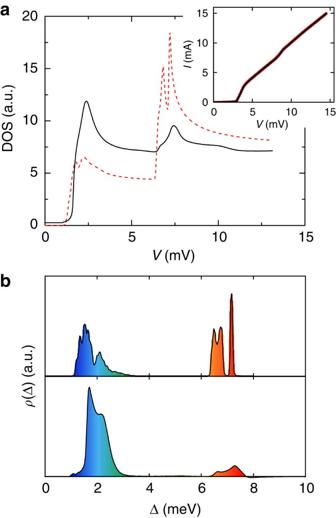Figure 3: The density of states and energy gap distribution of MgB2. (a) The superconducting DOS of MgB2atT=0 as derived from the tunnellingI–Vcurve (solid line) and calculated (dashed line) from ref.1(inset). The tunnellingI–Vcurve atT=1.8 K as measured (black line) and reconstructed (red squares) from the derived distribution of MgB2energy-gap values. (b) The distribution of MgB2energy-gap values atT=1.8 K derived from the superconducting DOS (bottom) compared with the theoretical results (top) of ref.1. The MgB 2 DOS is shown in Figure 3a, together with the DOS, calculated by Choi et al . [1] The gap distribution ρ (Δ) is related to the DOS by the relation The gap distribution found by deconvoluting the DOS is shown in Figure 3b . The validity of the deconvolution algorithms is justified by the overlap between the experimental I – V curve and the reconstructed I – V curve from the derived ρ (Δ), as shown in the inset of Figure 3a . Figure 3: The density of states and energy gap distribution of MgB 2 . ( a ) The superconducting DOS of MgB 2 at T =0 as derived from the tunnelling I – V curve (solid line) and calculated (dashed line) from ref. 1 (inset). The tunnelling I – V curve at T =1.8 K as measured (black line) and reconstructed (red squares) from the derived distribution of MgB 2 energy-gap values. ( b ) The distribution of MgB 2 energy-gap values at T =1.8 K derived from the superconducting DOS (bottom) compared with the theoretical results (top) of ref. 1 . 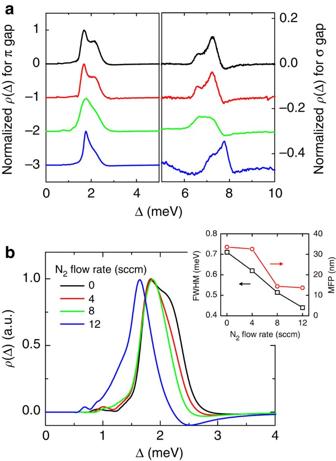Figure 4: Variation in the energy gap distribution in different MgB2junctions. (a) The energy gap distributions for four junctions: A (black), B (red), C (Green) on MgO (211) and D (blue) onc-axis-8°-tilted SiC. Each curve is normalized to its peak value and shifted vertically for clarity. Curves for junctions A and C were obtained atT=1.8 K and those for junctions B and D were obtained atT=4.2 K. The values of the productRnAare 1.6, 0.82, 7.7 and 2.6 mΩcm2for junctions A, B, C and D, respectively. The σ-gap curve for junction D is magnified five times. (b) The energy gap distribution around π gap region for 4 junctions on SiC (0001) substrates atT=4.2 K with different N2flow rates during the MgB2growth. (inset) The dependence of FWHM of the gap distribution peaks and the electron mean free path (MFP) to the flow rate of N2addition. Full size image Effects of electron scattering on gap features In Figure 4a , the gap distribution normalized to the peak value of ρ (Δ) is shown for several other MgB 2 /native oxide/Pb junctions on different substrates. The R n A product, where R n is the junction normal-state resistance and A is the junction area, ranges from 0.82 to 7.7 mΩcm 2 . As the intraband scattering rate in the MgB 2 electrode is very sensitive to details of the deposition conditions, it varies from junction to junction [20] . As a result, the fine structures in the gap distributions are more distinct in some junctions than in others. Because of epitaxial tensile strain [21] , MgB 2 films on SiC substrates have higher T c s (over 41 K) than films on MgO substrates (about 38.3 K), and consequently the average σ gap is larger. To vary the scattering rate systematically, N 2 gas (99.999% purity) was added to the carrier gas during the MgB 2 deposition, since the trace amount of oxygen in N 2 leads to scattering centres in the MgB 2 films [22] . Figure 4b shows the π peaks in ρ (Δ) for four junctions on SiC (0001) substrates with different flow rates of N 2 addition. As seen in the inset, the electron mean free path, derived from the electrical resistivity, becomes shorter and the energy distribution peak of the π gap becomes sharper (smaller FWHM) with increasing amounts of N 2 addition. This indicates that the intraband scattering smears out the gap distribution. Collectively, the results shown in Figure 4a,b indicate that the observed gap values and their distributions are sensitively affected by the electronic scattering in the MgB 2 films. Figure 4: Variation in the energy gap distribution in different MgB 2 junctions. ( a ) The energy gap distributions for four junctions: A (black), B (red), C (Green) on MgO (211) and D (blue) on c -axis-8°-tilted SiC. Each curve is normalized to its peak value and shifted vertically for clarity. Curves for junctions A and C were obtained at T =1.8 K and those for junctions B and D were obtained at T =4.2 K. The values of the product R n A are 1.6, 0.82, 7.7 and 2.6 mΩcm 2 for junctions A, B, C and D, respectively. The σ-gap curve for junction D is magnified five times. ( b ) The energy gap distribution around π gap region for 4 junctions on SiC (0001) substrates at T =4.2 K with different N 2 flow rates during the MgB 2 growth. (inset) The dependence of FWHM of the gap distribution peaks and the electron mean free path (MFP) to the flow rate of N 2 addition. Full size image The gap distribution derived from the tunnelling spectrum is in agreement with the first-principles calculations [1] , [2] . Both the π and σ gaps split into several peaks with the peak positions similar to those predicted by Choi et al . [1] as can be seen from Figure 3b . The spread in values for the π gap is 2.3 meV and is 1.3 meV for the σ gap, which are close to the spreads predicted by Choi et al .. The results are also compatible with preliminary superconducting density functional theory calculations by Massidda, Sanna, and Profeta (personal communication) performed with a full k -space resolution. As different groups are using different theoretical approaches to MgB 2 and have produced differing values of the electron–phonon coupling coefficients, our results can be used to facilitate experimental verification of theories. The magnitudes of peaks for 6 meV<Δ σ <8 meV are much smaller than for the range 1 meV<Δ π <3 meV, which is opposite to the theoretical predictions. (Similar discrepancies are seen in the DOS shown in Fig. 3a .) The most probable reason is that, in our junctions, the σ-band charge carriers account for only 11% of the total tunnel current, whereas the theoretical result is effectively for isotropic tunnelling, where the σ-band contribution is around 33% (ref. 23 ). Mazin et al . have pointed out that the fine structure in the distribution of gaps cannot be experimentally observed unless the intraband scattering rate satisfies where ‹Δ› is the average gap value for the band and δΔ is the variation of the gap value for the band [14] . They estimated that the electron mean free path of the MgB 2 sample has to exceed 150 nm. Taking the values of ‹Δ› and δΔ from Figure 3b , the maximum intraband scattering rates in the MgB 2 film are estimated to be 0.9 and 1.7 meV for the π and σ bands, respectively. In the clean MgB 2 film grown by HPCVD, the mean free path can be as large as 280 nm (ref. 24 ), which is most likely the reason that the fine structure in the gap distributions becomes observable in our junctions. The sensitivity of the fine structure in the gap distribution to the scattering rate shown in Figure 4a and the smearing out of the structure by the increasing number of scattering centres shown in Figure 4b are all in agreement with the multiband theory of Mazin et al . [14] Another factor that can affect the fine structure in the gap distribution is the scattering at the superconductor/insulator interfaces, which may cause all the states in the σ or π bands to mix. Indeed, the fine structure is smeared out in junctions with large values of the product R n A , which, besides being due to thicker barriers, can also be partially due to strong interface scattering. It is not clear whether further fine structure will be observed if the scattering in MgB 2 is reduced, or whether the observed resolution in the gap distribution already represents the limit imposed by surface mixing of carriers in the bands with different momenta. In summary, we have studied tunnelling spectroscopy in MgB 2 /native oxide/Pb tunnel junctions and have found a distribution of the superconducting gap values for the σ and π bands in MgB 2 . This is possible because the MgB 2 electrode grown by HPCVD was clean and had a long mean free path. In dirty single-band superconductors, the energy gap is single-valued because the scattering smears out the momentum dependence of the electron–phonon interaction [25] . For dirty MgB 2 samples, both the σ and π gaps are single-valued owing to the effect of intraband scattering, but they remain distinct from each other because the interband scattering rate is small owing to the disparity of electronic structure of the two bands [26] . When the MgB 2 sample is clean, the distribution of the energy-gap values becomes important. One dramatic consequence of the gap distribution is the smearing of the DOS singularity at the gap ( Fig. 3a ) and the absence of a sharp rise in current in the I - V curves of tunnel junctions (inset of Fig. 3a ). These are properties of clean superconductor junctions that must be confronted when considering their applications [27] . Fabrication of tunnel junctions To fabricate the MgB 2 /native oxide/Pb junctions, a 100-nm thick MgB 2 bottom electrode layer was first epitaxially grown on a MgO (211), SiC (0001), or c -axis-8°-tilted SiC substrate by HPCVD. Because of the high purity of the Mg and B sources and the reducing hydrogen atmosphere during the deposition, MgB 2 films, prepared by HPCVD, are exceptionally clean [24] , [28] . The mean free path of the MgB 2 films, as estimated by the residue resistivity, can be greater than 280 nm and, in our case, is limited by the thickness of the film (~100 nm) [29] . The transition temperature T c of the MgB 2 films on MgO substrates is around 38.3 K and is 41.2 K on SiC substrates. To vary the scattering rate in MgB 2 films, N 2 gas (99.999% purity) with flow rate from 0 to 12 sccm (standard cubic centimetres per minute) was introduced along with 1,200 sccm H 2 and 20 sccm B 2 H 6 (5% in H 2 ) during the MgB 2 growth. The MgB 2 film was then exposed to air at room temperature to form a native oxide barrier [30] . The bottom electrode stripe was subsequently created by painting the sample with Duco Cement. The 200-nm-thick Pb top electrode stripes, orthogonal to the bottom electrode stripe, were formed by thermal evaporation through a shadow mask at a background vacuum of around 1×10 −5 mbar. The junction size was about 0.3 mm×0.3 mm. Tunnelling spectra measurements Four-probe electrical measurements were carried out in a Physical property measurement system at temperatures down to 1.8 K. During the measurement, an in-plane magnetic field up to 1 mT was applied to suppress the Josephson current. The tunnelling I – V curves were acquired in current-bias mode and the tunnelling conductance d I /d V – V curves were acquired by a lock-in amplifier with a 262 Hz 50 μV root-mean-square modulation applied to the sample. The integration time constant was 1 s with a bias sweep rate outside the π gap of about 20 μV s −1 . How to cite this article: Chen, K. et al . Momentum-dependent multiple gaps in magnesium diboride probed by electron tunnelling spectroscopy. Nat. Commun. 3:619 doi: 10.1038/ncomms1626 (2012).